Three-dimensional broadband and broad-angle transformation-optics lens Luneburg lenses have superior performance compared with conventional lenses made of uniform materials with specially designed surfaces, but they are restricted by the difficulty of manufacturing the required gradient-index materials and their spherical focal surfaces. Recently, a new two-dimensional (2D) imaging lens was proposed and realized using transformation optics. Such a 2D lens overcomes the aberration problem, has a flattened focal surface and is valid for extremely large viewing angles. Here, we show the design, realization and measurement of a three-dimensional (3D) approximate transformation-optics lens in the microwave frequency band. The 3D lens is made of non-resonant metamaterials, which are fabricated with multilayered dielectric plates by drilling inhomogeneous holes. Simulation and experimental results demonstrate excellent performance of the 3D lens for different polarizations over a broad frequency band from 12.4 to 18 GHz. It can also be used as a high-gain antenna to radiate or receive narrow beams in large scanning angles. Imaging is one of the most important activities in science and daily life. As imaging tools, optical lenses have been investigated by many scientists and industries for several centuries. In a conventionally positive or converging lens, made of a uniform material (such as the glass or transparent plastic) with a specially designed surface, a collimated beam travelling along the lens axis is focused to a spot, the focal point, at a distance f (known as the focal length) from the lens, or a point source at the focal point is converted into a collimated beam by the lens. Hence, an object at an infinite distance is focused to an image at the focal point, or an object at the focal point has an image at infinity. As the focusing principle of the conventional lens is based on the refraction of light rays on the lens surface and the straight-line transmission inside the lens, there always exist geometrical and wave aberrations (such as spherical aberration, coma, chromatic aberration and so on) that limit the imaging quality of the conventional lenses. Although multiple optimized lenses can be used to form a lens array, imaging distortion due to aberration is still unavoidable. The other type of lenses, which are composed of inhomogeneous materials with radially decreasing refractive indices and are known as Luneburg lenses, can eliminate the aberration. A Luneburg lens is a spherical lens that generates perfect geometrical images of two given concentric spheres onto each other. There are an infinite number of refractive index solutions to Luneburg lenses to determine different focusing properties, and the simplest one is given by n =(2− r 2 / R 2 ) 1/2 , in which R is the radius of the sphere [1] . In such a Luneburg lens, if one focal point lies at infinity, the other one will be on the opposite surface of the lens. Hence, the gradient index of refraction inside the Luneburg lens guides the incoming collimated rays from infinity to a focal point on the spherical surface without any aberrations. The practical Luneburg lens is normally realized using layered concentric shells with different refractive indices, forming a stepped refractive index profile to approximate the gradient one. Such implementation is usually used in the microwave frequency to construct microwave antennas, but it is hardly used in the optical frequency band. Recently, non-resonant metamaterials have been applied to build the 2D Luneburg lens antenna in the microwave frequency [2] . Besides the difficult fabrication challenge of the required gradient-index materials, the other restriction of Luneburg lens is the spherically focal surface, which cannot be well matched to the planar feeding source or detector array. To overcome the restriction, a significant achievement has been made by generating a novel metamaterial lens based on the Luneburg lens [3] , [4] . Using the transformation optics [4] , [5] , the circularly focal surface can be changed as a flattened focal plane, and the incoming collimated rays from extremely large angles can all be focused to this plane [3] , [4] . Compared with the conventional uniform material lens and the circular Luneburg lens, the new lens has no aberration, a zero focal distance (a focal distance is defined as the distance from the focal point to the lens), a flattened focal surface and the ability to form images at extremely large angles. Hence, such a kind of lens could be a good candidate for high-quality imaging applications. A prototype of the new lens was demonstrated using metamaterial structures in the microwave region over a broadband [3] . However, this demonstration was only limited to a 2D form with the transverse electric mode. In this work, we present the design, realization and measurement of a 3D version of the 2D transformation-optics lens in the microwave frequency. This is actually an approximate 3D transformation-optics lens, which is composed of non-resonant metamaterials and fabricated with multilayered isotropic dielectric plates by drilling inhomogeneous holes. Simulation and experimental results demonstrate excellent performance of the 3D lens with low loss for different polarizations over a broad frequency band from 12.4 to 18 GHz (Ku-band), which can be used as a high-gain antenna with narrow beams and large scanning angles. Design of the 3D transformation-optics lens In the design of the new 3D lens, transformation optics has an important role. It has been widely used to design and generate other attractive devices such as invisibility cloaks [5] , [6] , [7] , [8] , [9] , [10] , [11] , [12] , [13] , [14] , [15] , [16] , electromagnetic concentrators and rotators [17] , [18] , [19] and high-performance antennas [20] , [21] . 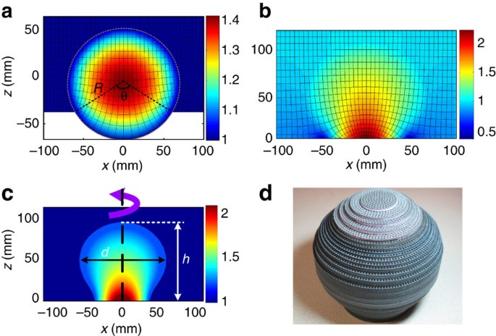Figure 1: Quasi-conformal mapping of 2D flattened Luneburg lens and generation of 3D flattened Luneburg lens. (a) The 2D Luneburg lens and its transformation space, in whichR=70 mm andθ=120°. (b) The 2D flattened Luneburg lens and its refractive index distribution. (c) The simplified refractive index distribution in thexozplane. The 3D lens is generated by rotating the profile around thezaxis. (d) The photograph of the fabricated 3D lens. To design the 3D Luneburg-based lens, we start from a 2D geometry shown in Figure 1. The virtual space is a Luneburg surface with a radius R and the normal refractive index distribution ( n= (2– r 2 / R 2 ) 1/2 ) in the free space ( Fig. 1a ). We intended to flatten a part of the circular surface with an open angle θ , as shown in Figure 1a . If θ= 180°, half of the circular surface will be flattened. Hence, the physical space is illustrated in Figure 1b , which is a rectangular region. Transformation from the virtual space to the physical space can be performed using two approaches. The first approach is the exact coordinate transformation, which results in strongly anisotropic metamaterials in the physical space [4] . Hence, the approach is difficult to realize in experiments. The other approach is based on quasi-conformal mapping [3] , [7] , which numerically generates the spatial transformation. In this method, only isotropic dielectric materials are required in the physical space [3] , which are much easier to realize in experiments. Figure 1: Quasi-conformal mapping of 2D flattened Luneburg lens and generation of 3D flattened Luneburg lens. ( a ) The 2D Luneburg lens and its transformation space, in which R =70 mm and θ =120°. ( b ) The 2D flattened Luneburg lens and its refractive index distribution. ( c ) The simplified refractive index distribution in the x o z plane. The 3D lens is generated by rotating the profile around the z axis. ( d ) The photograph of the fabricated 3D lens. Full size image We adopt the second approach in our design and set the open angle as θ =120° ( Fig. 1a ). The quasi-conformal mapping result is shown in Figure 1b , from which we clearly see that the range of refractive index varies from 0.5 to 2.2. We also notice that only a small portion in the physical space is occupied by materials the refractive index of which is less than 1 ( n <1). Although such materials could be realized using metamaterials near the resonant frequency, the large loss and narrow bandwidth will restrict the overall performance of the novel lens. Hence, we make an approximation in the design and experiments to replace the small portion ( n <1) by free space ( n =1). After such an approximation, the final 2D refractive index profile in the x o z plane is illustrated in Figure 1c , the index of refraction of which is varied from 1.1 to 2.1. We generate the 3D refractive index distribution by rotating the 2D profile along the z axis ( Fig. 1c ). In this manner, a novel 3D Luneburg lens is achieved, as shown in Figure 1d , in which the z axis is called the optical axis and the x o y plane is the focal surface. From Figure 1a , the 3D lens has a height of h =104 mm and a maximum aperture of d =108 mm. As presented in Methods, this is an approximate transformation-optics lens [22] . When a source is placed at different positions on the flattened focal surface, the lens will radiate perfectly planar wavefronts at different angles on the planes containing the optical axis. On the planes not containing the optical axis, the planar wavefronts will have some distortions. Performance simulation To illustrate the performance of the approximate 3D transformation-optics lens, we generate full-wave simulations using commercial software (Microwave Studio, CST). The simulation model is generated from Figure 1c by rotating the 2D profile along the z axis, as demonstrated in Supplementary Figure S1 . The feeding source is a rectangular waveguide (aperture size: 16 × 8 mm 2 ), which is the same as that used in experiments. When the feed is located at the centre of the focal plane ( x =0 and y =0), the simulation results of the near-field distributions on yz planes (vertical planes) are shown in Supplementary Figure S2 , in which a–c illustrate the electric fields on the x =0 plane (containing the optical axis) at different frequencies of 12.5, 15 and 18 GHz, and d, e demonstrate the fields on planes x =10, 30 and 40 mm at 15 GHz. From a–c, we clearly observe that the 3D lens produces perfectly planar wavefronts in a broad frequency band on the plane containing the optical axis, as predicted; from d, e, surprisingly, we observe nearly perfect planar wavefronts on planes not containing the optical axis, even when the plane is far away from the optical axis ( x =40 mm, which is close to the edge of the lens). Similar phenomena are observed on the horizontal planes ( xz planes), as shown in Supplementary Figure S3 . 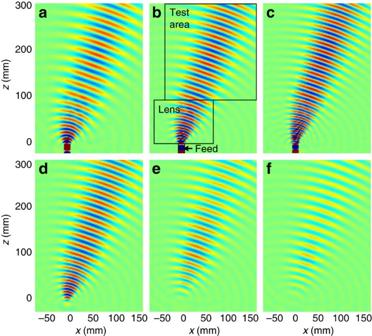Figure 2: Simulated near-field distributions of the 3D lens. Here, the feeding source is located 10 mm off the centre of the focal plane (x=−10 mm andy=0). (a–c) On they=0 plane (containing the optical axis) at 12.5, 15 and18 GHz. (d–f) Ony=10, 30 and 40-mm planes at 15 GHz. When the feed moves a short distance from the centre of the focal plane ( x =−10 mm and y =0), the near-field distributions on the horizontal in-optical-axis plane ( y= 0) at 12.5, 15 and 18 GHz are illustrated in Figure 2a–c ; and field distributions on the off-optical-axis plane ( y= 10, 30 and 40 mm) at 15 GHz are shown in Figure 2d,e . Obviously, the 3D lens also produces nearly perfect planar wavefronts on both planes containing and not containing the optical axis, directing to the angle of 20° off the z axis. 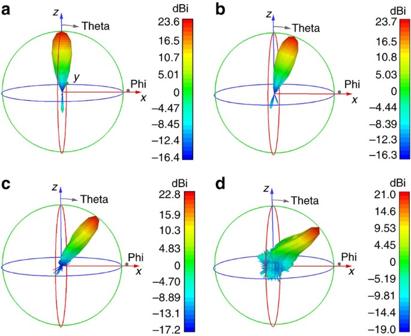Figure 3: Simulated 3D far-field radiation patterns of the 3D lens at 15 GHz. (a) The feeding source is located at the centre of the focal plane (x=0 andy=0). (b–d) The feeding source is located 10, 20 and 30 mm off the centre of the focal plane (x=−10, −20 and −30 mm, andy=0). Owing to the good planar wavefronts in 3D space, the lens can serve as a high-gain and low-sidelobe antenna, which can be clearly seen in the 3D far-field radiation patterns depicted in Figure 3a,b . Figure 2: Simulated near-field distributions of the 3D lens. Here, the feeding source is located 10 mm off the centre of the focal plane ( x =−10 mm and y =0). ( a – c ) On the y =0 plane (containing the optical axis) at 12.5, 15 and18 GHz. ( d – f ) On y =10, 30 and 40-mm planes at 15 GHz. Full size image Figure 3: Simulated 3D far-field radiation patterns of the 3D lens at 15 GHz. ( a ) The feeding source is located at the centre of the focal plane ( x =0 and y =0). ( b – d ) The feeding source is located 10, 20 and 30 mm off the centre of the focal plane ( x =−10, −20 and −30 mm, and y =0). Full size image As the feed moves a relatively large distance from the centre of the focal plane ( x =−20 mm and y =0), the simulation results on near and far fields are demonstrated in Supplementary Figures S4 and S3c . In this situation, the planar wavefronts only have small distortions on the observation planes that are far from the optical axis ( y= 30 and 40 mm), which still result in a very good radiating beam to the angle 37° off the z axis. As the feed reaches the boundary of the focal plane ( x =−30 mm and y =0), the electric field distributions on the in-optical-axis plane ( y= 0) and the nearby off-optical-axis plane ( y= 10 mm) demonstrate very good planar wavefronts, making a large radiation angle of 50° ( Supplementary Fig. S5a–d ). Only when the observation planes are far from the optical axis ( y= 30 and 40 mm) do the field patterns have severe distortions ( Supplementary Fig. S5e,f ). However, the far-field radiation pattern is still fair, as shown in Figure 3d . Hence, the approximate 3D transformation-optics lens has a very good overall performance, although small distortions exist near the edge of the lens. Realization of the 3D transformation-optics lens The 3D lens is composed of non-resonant metamaterials, which are fabricated with multilayered dielectric plates, and each layer is drilled by different inhomogeneous holes to realize the 3D distribution of refractive indices ( Fig. 1c ). Figure 1d illustrates the photograph of the final sample of the 3D lens. Two kinds of dielectric plates are involved in the lens' realization: the FR4 dielectric, which has a large relative permittivity 4.4 (with loss tangent 0.025), and the F4B dielectric, which has a small relative permittivity 2.65 (with loss tangent 0.001). We design the 3D transformation-optics lens to work in the Ku-band (the frequency ranges from 12.4 to 18 GHz), and choose three kinds of unit cells as building blocks of metamaterials to achieve the required distribution of refractive index. The three kinds of unit cells are 2 × 2× 1 ( Fig. 4b ) and 2 × 2× 2 mm 3 F4B dielectric blocks ( Fig. 4c ), and 2 × 2 × 2 mm 3 FR4 dielectric blocks ( Fig. 4d ), which can be easily generated from the commercial 1-mm-thick and 2-mm-thick F4B plate, and 2-mm-thick FR4 plate, respectively. The continuous variation of the refractive index ( n ) can be obtained by changing the diameter ( D ) of the drilling hole in the unit cell. 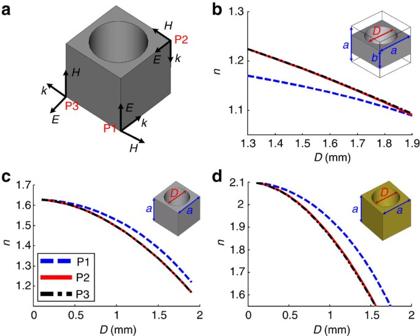Figure 4: Relations between the refractive index and the hole's diameterD.These relations are shown for different unit cells under different polarizations at 15 GHz. (a) Three polarizations P1, P2 and P3 for a unit cell, (b) the 2 × 2 × 1 mm3F4B unit cell, (c) the 2 × 2 × 2 mm3F4B unit cell and (d) the 2 × 2× 2 mm3FR4 unit cell. Figure 4: Relations between the refractive index and the hole's diameter D. These relations are shown for different unit cells under different polarizations at 15 GHz. ( a ) Three polarizations P1, P2 and P3 for a unit cell, ( b ) the 2 × 2 × 1 mm 3 F4B unit cell, ( c ) the 2 × 2 × 2 mm 3 F4B unit cell and ( d ) the 2 × 2× 2 mm 3 FR4 unit cell. Full size image From the effective medium theory [23] , [24] and the S-parameter retrieval method [25] , effective indices of refraction for the above unit cells have been obtained, as demonstrated in Figure 4b–d . Here, three orthogonal polarizations of incident waves (P1, P2 and P3; Fig. 4a ) are considered for the study of the isotropic properties of unit cells. We observe that all three kinds of unit cells have nearly the same electromagnetic responses to P2- and P3-polarized incident waves and a slightly different response to the P1-polarized wave. Hence, all unit cells are approximately isotropic. For the 2 × 2 × 1 mm 3 F4B unit cell, the refractive index n changes from 1.23 to 1.08 as diameter D varies from 1.3 to 1.9 mm ( Fig. 4b ); for the 2 × 2 × 2 mm 3 F4B unit cell, n changes from 1.63 to 1.17 as D varies from 0.1 to 1.9 mm ( Fig. 4c ); and for the 2 × 2× 2 mm 3 FR4 unit cell, n changes from 2.1 to 1.56 as D varies from 0.1 to 1.7 mm ( Fig. 4d ), covering all required indices of refraction. In realization, the first region of 3D lens (the top part, Supplementary Fig. 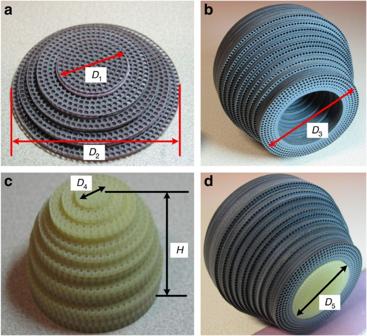Figure 5: Construction of the 3D transformation-optics lens. Here,D1=26 mm,D2=66 mm,D3=70 mm,D4=10 mm,D5=46 mm andH=40 mm. (a) The first region (the top part) was fabricated using 2 × 2 × 1 mm3F4B unit cells. (b) The second region (the bottom shell) was fabricated using 2 × 2 × 2 mm3F4B unit cells. (c) The third region (the bottom core) was fabricated using 2 × 2 × 2 mm3FR4 unit cells. (d) Construction of the 3D lens. S6d ), the refractive index of which changes from 1.1 to 1.2, was fabricated using 2 × 2 × 1 mm 3 F4B unit cells with different-sized holes, as shown in Figure 5a . Here, an additional 1-mm-thick foam plate, the refractive index of which is nearly 1, was placed under the 2 × 2 × 1 mm 3 F4B unit cells to achieve the same height as the 2 × 2 × 2 mm 3 unit cells for easy assemblage of the 3D lens. In the second region (the bottom shell; Supplementary Fig. S6d ), the refractive index varies from 1.2 to 1.63, and hence it can be fabricated using 2 × 2 × 2 mm 3 F4B unit cells with different-sized holes, as shown in Figure 5b . The third region is the bottom core, which has a large index of refraction (from 1.63 to 2.1), and hence was realized by 2 × 2 × 2 mm 3 FR4 unit cells with different-sized holes, as demonstrated in Figure 5c . The whole 3D lens was achieved by fixing the three parts together, as depicted in Figure 5d . The detailed fabrication process of the 3D lens is given in Supplementary Figure S6 . Figure 5: Construction of the 3D transformation-optics lens. Here, D 1 =26 mm, D 2 =66 mm, D 3 =70 mm, D 4 =10 mm, D 5 =46 mm and H =40 mm. ( a ) The first region (the top part) was fabricated using 2 × 2 × 1 mm 3 F4B unit cells. ( b ) The second region (the bottom shell) was fabricated using 2 × 2 × 2 mm 3 F4B unit cells. ( c ) The third region (the bottom core) was fabricated using 2 × 2 × 2 mm 3 FR4 unit cells. ( d ) Construction of the 3D lens. Full size image Experimental results To verify the actual performance of the 3D transformation-optics lens, we measured both near and far electric fields produced by the lens when a feeding source is placed at different positions on the flattened focal surface. 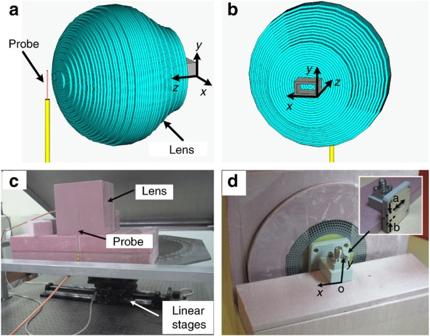Figure 6: Near-field measurement system of the 3D lens. (a–b) Demonstration of the relationship among probe, feed and lens. (c) A coaxial probe was used to detect the electric fields on a horizontal plane. (d) A Ku-band coax-to-waveguide device with the aperture size of 16 × 8 mm2was used to feed the lens at different positions on the flattened focal surface. The near-field measurement setup is illustrated in Figure 6 . A coaxial probe was placed in front of the lens ( Fig. 6a,c ) to detect the electric fields in the near-field region. The measured plane in experiments is on the x o z plane with y =0 mm ( Fig. 6a ), which contains the optical axis. The test region is a 198 × 198 mm 2 square area outside the 3D lens, which is shifted when the feeding source is placed at different locations, as shown in the square frames in Supplementary Figures S3b and S5b , and Figure 2b . A Ku-band coax-to-waveguide device with an aperture size of 16 × 8 mm 2 ( a =16 mm, b =8 mm) was used to feed the antenna (the feeding source; Fig. 6b,d ). In experiments, the 3D lens was fixed into a foam box for easy installation ( Fig. 6c ). The foam has a refractive index of nearly 1, and hence has little effect on measurements. The detection probe was fixed, and the 3D lens was controlled by an electronic motor under an aluminium plate that moves automatically to measure the near fields continuously, as shown in Figure 6c . From the ray trace analysis [22] and full-wave numerical simulations ( Figs 2 and 3 ; Supplementary Figs S2 , S3 , S4 , S5 ), the 3D lens will generate collimated rays (or plane waves) with small distortions, propagating to different directions by changing the feeding source positions. We remark that the detection probe should be parallel to the polarization direction of electric fields to get the best measurement results. Different polarizations in measurements can be considered by adjusting the feeding coax-to-waveguide device. When side a of the feed is parallel to the x axis (horizontally placed; Fig. 6 ), it corresponds to vertical polarization (to electric field); when side a of the feed is parallel to the y axis (vertically placed), it corresponds to horizontal polarization. Figure 6: Near-field measurement system of the 3D lens. ( a – b ) Demonstration of the relationship among probe, feed and lens. ( c ) A coaxial probe was used to detect the electric fields on a horizontal plane. ( d ) A Ku-band coax-to-waveguide device with the aperture size of 16 × 8 mm 2 was used to feed the lens at different positions on the flattened focal surface. 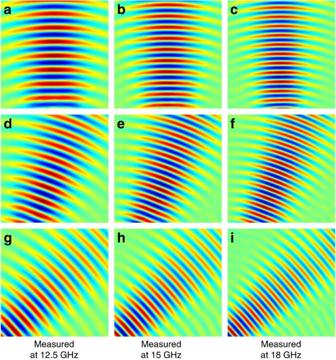Figure 7: Measurement results of near electric fields outside the 3D lens. The measurements are shown at 12.5, 15 and 18 GHz. (a–c) The feeding source is located at the centre of the focal plane (x=0 andy=0). (d–f) The feeding source is 10 mm off the centre of the focal plane (x=−10 mm andy=0). (g–i) The feeding source is 30 mm off the centre of the focal plane (x=−30 mm andy=0). Full size image The measurement results of the near electric fields under vertical polarization are illustrated in Figure 7 , in which three typical source positions are chosen on the focal plane: the feed is located at the lens centre ( x =0 and y =0; Fig. 7a–c ), 10 mm off the lens centre ( x =−10 mm and y =0; Fig. 7d–f ) and 30 mm off the lens centre ( x =−30 mm and y =0; Fig. 7g–i ). Such settings are the same as those in the full-wave simulations for fair comparison. In measurements, the electric fields inside the 3D lens cannot be obtained and the measurement region is marked as square frames in Figure 2b and Supplementary Figures S3b and S5b . Comparing Figure 7a–c with Supplementary Figure S3a–c ; Figure 7d–f with Figure 2a–c; and Figure 7g–i with Supplementary Figure S5a–c , we clearly notice that the measurement results have excellent agreement with the numerical simulations at all frequencies. More specifically, when the feed is located at the centre of the focal plane, the 3D lens generates very good planar wavefronts in the z direction ( Fig. 7a–c ); when the source is 10 mm off the centre ( x =−10 mm and y =0), the 3D lens radiates good plane waves propagating in the angle of 20° off the z direction ( Fig. 7d–f ); as the source is 30 mm off the centre ( x =−30 mm and y =0), the plane waves propagate in the direction of 50° off the z axis ( Fig. 7g–i ). The simulated and measured radiation angles have a perfect match. As the 3D lens was fabricated using multilayer isotropic dielectric plates by drilling inhomogeneous holes, the lens works in a broad frequency band from 12.4 to 18 GHz. From the above measurement results, we clearly observe that the radiation direction can be controlled in a large angle range by moving the feeding source on the flattened focal surface in the whole Ku-band. Figure 7: Measurement results of near electric fields outside the 3D lens. The measurements are shown at 12.5, 15 and 18 GHz. ( a – c ) The feeding source is located at the centre of the focal plane ( x =0 and y =0). ( d – f ) The feeding source is 10 mm off the centre of the focal plane ( x =−10 mm and y =0). ( g – i ) The feeding source is 30 mm off the centre of the focal plane ( x =−30 mm and y =0). Full size image The 3D lens was also measured in the anechoic chamber to observe the far-field radiations in both horizontal and vertical polarizations. 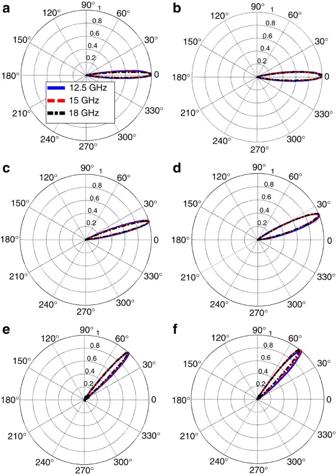Figure 8: Measured far-field results of the 3D lens. (a,c,e) Show horizontal polarizations, whereas (b,d,f) present vertical polarizations at 12.5, 15 and 18 GHz. (a–b) The feeding source is located at the centre of the focal plane (x=0 andy=0). (c–d) The feeding source is 10 mm off the centre of the focal plane (x=−10 mm andy=0). (e–f) The feeding source is 30 mm off the centre of the focal plane. The measured far-field radiation patterns are illustrated in Figure 8, with different feeding positions on the flattened focal surface at different frequencies. Figure 8a,c,e demonstrates the horizontally polarized (E-plane) far-field radiation patterns at 12.5, 15 and 18 GHz; and Figure 8b,d,f shows the vertically polarized (H-plane) far-field radiation patterns at 12.5, 15 and 18 GHz, respectively. To observe the sidelobe information clearly, we replot the far-field radiation patterns in the log scale (dB), as depicted in Supplementary Figure S7 . From Figure 8 and Supplementary Figure S7 , the broadband property of the 3D lens is well kept in the far-field radiations, which is valid for both horizontal and vertical polarizations. The main features of the 3D transformation-optics lens are given in Supplementary Table S1 . Apparently, it has very good overall performance. As a planar array of feeding sources is placed on the flattened focal surface, the radiation beam of the 3D lens will be scanned in a range of 50° with respect to the normal direction ( z axis). Figure 8: Measured far-field results of the 3D lens. ( a , c , e ) Show horizontal polarizations, whereas ( b , d , f ) present vertical polarizations at 12.5, 15 and 18 GHz. ( a – b ) The feeding source is located at the centre of the focal plane ( x =0 and y =0). ( c – d ) The feeding source is 10 mm off the centre of the focal plane ( x =−10 mm and y =0). ( e – f ) The feeding source is 30 mm off the centre of the focal plane. Full size image In the last 10 years, metamaterials have received great attention because of their unusual properties and behaviours. However, most metamaterial research is still limited to theory and numerical simulations, and only a few experiments have been performed. Among the limited metamaterial experiments, most of them have been restricted to 2D cases except the recently proposed 3D ground plane invisibility cloaks [15] , [16] . Even for the 3D invisibility cloaks, there is still a long way to find real applications because of their large sizes compared with cloaked objects. In this article, we have demonstrated the design, realization and measurement of a novel 3D lens in the microwave frequency. This is the first 3D lens based on transformation optics, although it is an approximation. Hollowed dielectric plates are used to build the 3D lens, which are easy to realize and could be popularized in the scientific community. The proposed 3D lens is more advantageous than conventional uniform material lens and the spherical Luneburg lens, with zero focal distance, flattened focal surface and ability to generate radiation beams at extremely large angles. The ray trace analysis [22] and full-wave numerical simulations show that the 3D lens can radiate perfectly planar wavefronts on planes containing the optical axis no matter where the feeding source is located and how large the radiation angle is, which has also been confirmed by experiments. As the feeding source is located near the centre of the focal plane, very good planar wavefronts are observed on all planes not containing the optical axis. When the feeding source is far away from the centre and close to the edge of the focal plane, the planar wavefronts are well kept on planes not containing but close to the optical axis. Only on planes far away from the optical axis do the wavefronts have severe distortions. Hence, the 3D lens has very good overall performance: (1) high gain; (2) relatively low sidelobes (especially for small radiation angles); (3) dual polarizations; (4) large radiation angles (up to 50°); and (5) broad band (from 12.4 to 18 GHz). If a planar array of feeding sources is placed on the flattened focal surface and is properly controlled, the radiation beam will be scanned in a range of 50° around the z axis, realizing a high-performance beam-scanning antenna. The above performance makes the novel 3D lens superior than traditional antennas, as presented in Methods. Approximation of the 3D transformation-optics lens Although the 2D profile shown in Figure 1c is obtained using quasi-conformal mapping, it was demonstrated that the rotational 3D distribution of the refractive index does not satisfy the requirement of the optical transformation [22] . From the rigorous analysis, an accurate 3D transformation-optics lens should be made of anisotropic materials with both electric permittivity and magnetic permeability tensors [22] . This can be clearly seen from the local dispersion relation for the cylindrical coordinate system ( ρ , ϕ , z ), in which x 2 + y 2 = ρ 2 and tan ϕ=y / x . The local dispersion relation has been derived as [22] in which is the normalized wavenumber with respect to free space, α = ɛ ϕ , β 2 = ɛ ρ =ɛ z , and ( ɛ ρ , ɛ ϕ , ɛ z ) are permittivity components of the anisotropic materials. Only when k ϕ =0 does the above equation reduce to the dispersion relation for an isotropic dielectric medium ( ɛ = α ). Hence, the proposed 3D lens that is composed of isotropic dielectric materials is an approximate transformation-optics lens, which is accurate only when k ϕ =0. Under the condition of cylindrical symmetry of the proposed 3D lens, k ϕ =0 implies constant ϕ planes, or the planes containing the optical axis. As a consequence, all incident rays on the planes containing the optical axis at a wide range of angles can be focused onto the flattened focal surface, which is exactly the same as the 2D case [3] . If the rays impinge on planes not containing the optical axis, however, they cannot be exactly focused. On the other hand, when a source is placed at different positions on the flattened focal surface, the lens will radiate perfectly planar wavefronts at different angles on the planes containing the optical axis. On the planes not containing the optical axis, the planar wavefronts will have some distortions. Performance comparison with traditional antennas It is hard to find an appropriate traditional antenna to make full comparisons with the 3D transformation-optics lens. For example, the phase-array antenna is a good candidate to scan large radiation angles [26] , but it requires an extremely complicated feeding network with very high cost; the leaky-wave antenna is restricted by its small scanning angles [26] ; and so on. To make fair comparisons, we choose a uniform material hyperbolic lens antenna [27] ( Supplementary Fig. S8a ) and a parabolic reflector antenna [27] ( Supplementary Fig. S8b ) that have the same aperture size (108-mm diameter) and are fed by the same waveguide (16 ×8 mm 2 ), because they also have the good performance of high gains, broadband and dual polarizations. The focal distances of the two antennas are 90 and 80 mm. When the feed moves on the focal plane, the radiation beams of the two antennas can also be scanned in a range of angles. The near-field distributions of the two traditional antennas are simulated using the same commercial software (Microwave Studio, CST), as illustrated in Supplementary Figure S9 . When the feed is located at the centre of the focal plane ( x =0), the two antennas radiate planar wavefronts to the normal direction ( z axis; Supplementary Fig. S9a,d ). As the feed is located 20 mm off the centre of the focal plane ( x =−20 mm), the hyperbolic lens radiates planar wavefronts to an angle of 10.5° off the z direction ( Supplementary Fig. S9b ), and the parabolic reflector radiates distorted planar wavefronts to an angle of 13.4° off the z direction ( Supplementary Fig. S9e ). When the feed is located at the edge of the focal plane ( x =−40 mm), the hyperbolic lens radiates planar wavefronts to an angle of 20.4° off the z direction ( Supplementary Fig. S9c ), and the parabolic reflector radiates distorted planar wavefronts to an angle of 21.1° off the z direction ( Supplementary Fig. S9f ). Hence, the maximum scanning angles for such two antennas are 20.4° and 21.1°, which are much smaller than that of the 3D flattened Luneburg lens (50°). We have also made comparisons for the far-field radiation patterns in horizontal polarization among the three antennas—the 3D transformation-optics lens, the hyperbolic lens and the parabolic-reflector antenna—at 15 GHz, as demonstrated in Supplementary Figure S10 . Supplementary Figure S10a shows the case when the feeding source is located at the centre of the focal plane ( x =0 and y =0), and Supplementary Figure S10b shows another case as the feeding source is located 10 mm off the centre of the focal plane ( x =−10 mm and y =0) for the new 3D lens and 40 mm off the centre of the focal plane ( x =−40 mm and y =0) for two traditional antennas. In the latter case, the radiation angles of all three antennas are around 20°. The comparison of the main features among the three antennas is given in Supplementary Table S2 . Clearly, the approximate 3D transformation-optics lens has much superior overall performance than the two traditional antennas. How to cite this article: Ma, H. F. & Cui, T.J. Three-dimensional broadband and broad-angle transformation-optics lens. Nat. Commun. 1:124 doi: 10.1038/ncomms1126 (2010).